Rare-earth-doped biological composites asin vivoshortwave infrared reporters The extension of in vivo optical imaging for disease screening and image-guided surgical interventions requires brightly emitting, tissue-specific materials that optically transmit through living tissue and can be imaged with portable systems that display data in real-time. Recent work suggests that a new window across the short-wavelength infrared region can improve in vivo imaging sensitivity over near infrared light. Here we report on the first evidence of multispectral, real-time short-wavelength infrared imaging offering anatomical resolution using brightly emitting rare-earth nanomaterials and demonstrate their applicability toward disease-targeted imaging. Inorganic-protein nanocomposites of rare-earth nanomaterials with human serum albumin facilitated systemic biodistribution of the rare-earth nanomaterials resulting in the increased accumulation and retention in tumour tissue that was visualized by the localized enhancement of infrared signal intensity. Our findings lay the groundwork for a new generation of versatile, biomedical nanomaterials that can advance disease monitoring based on a pioneering infrared imaging technique. Real-time, noninvasive optical imaging of diseases is limited by the availability of optical probes capable of being sensitively detected and rapidly resolved in living tissue while preferentially targeting features of clinical interest [1] . Probe detection is governed by emission intensity, optical path length through tissue and volumetric energy distribution, which are linked to the absorption and scattering properties of biological media and tissues [2] . Water, haemoglobin, melanin and lipids act as major absorbers of light, whereas the size, composition and morphology of biological tissues primarily scatter light [3] , [4] , [5] . Near infrared light (NIR, 700–1,000 nm) is absorbed less by tissue components than visible light [6] , resulting in greater penetration and thus deeper imaging [7] in the first ‘tissue-transparent window.’ Recently, optical simulations have led to predictions of a second ‘tissue-transparent window’ using short-wavelength infrared light (SWIR, 1,000–2,300 nm) with comparably low absorbance and tissue autofluorescence as NIR but up to a 1,000-fold greater reduction in scatter losses [2] , leading to unprecedented improvements in detection depth and resolution. Tissue-specific probes that can be detected using SWIR offer a means of utilizing this highly sensitive spectral ‘window’ to visualize pathological features that are not detected using conventional optical methods. However, widespread implementation of SWIR optical imaging for translational research has been hindered by a lack of bright and biocompatible probes [8] . Materials currently reported capable of generating SWIR emissions have significant limitations for biomedical applications including high toxicity and sub-optimal optical characteristics. SWIR-emitting semiconducting quantum dots (QDs) comprise toxic elements including lead, mercury and arsenic [9] , and therefore have not be used for in vivo imaging [10] . Although infrared-emitting single-walled carbon nanotubes (SWNTs) have been investigated for in vivo applications [11] , [12] , [13] , numerous challenges face the development of SWNTs as biomedical SWIR-imaging agents, most critically for multispectral and disease-targeted imaging. Owing to low quantum yield and optimal excitation outside the NIR–SWIR windows of transparency near 650 nm [11] , SWNTs require high-powered, pulsed excitation sources (>2 W) coupled with long camera exposure durations to achieve sufficient signal-to-background ratios for in vivo detection [14] . SWNTs also exhibit broad and low-intensity emission peaks spanning >300 nm [11] , preventing any practical tunability for multispectral imaging using non-overlapping signals. Furthermore, SWNTs have large length distributions spanning hundreds of nanometres [11] , [13] , which pose challenges for effectively addressing size-dependent biological barriers [15] . Ultimately, designing a successful SWIR-imaging probe must take into consideration the multiple parameters that influence the signal-to-background ratio including quantum yield, biodistribution, pharmacokinetics and target-site affinity as well as the in vivo toxicity and safety profiles of any new agent. [16] Recent evidence suggests that rare-earth nanomaterials (REs) are also capable of generating SWIR emissions with large Stokes shifts following excitation with low power, continuous wave sources in the NIR first ‘tissue-transparent window’ [17] . Traditionally, biomedical imaging using REs has relied on detecting the visible emissions that arise from NIR upconversion fluorescence ( Supplementary Fig. S1 ) [16] , [17] , largely ignoring the SWIR emissions simultaneously generated upon excitation. Therefore, an investigation into the SWIR-imaging properties of REs is necessary in order to assess the potential for these probes to be used as tools for visualizing biological features in vivo . Here we evaluate REs for in vivo SWIR imaging and provide the first demonstration of disease detection using a multispectral SWIR-imaging platform. We first develop a library of REs with tunable, discrete SWIR emissions and proceed to evaluate their optical performance for several clinical imaging applications including real-time, multispectral in vivo SWIR imaging. Our findings demonstrate that SWIR transmits more effectively through tissue phantoms than NIR light, and that imaging using REs offers superior detection sensitivity over other SWIR emitters. We further investigate the ability of REs to target and image malignancies by modifying the surface with human serum albumin (HSA). By controlling the thickness of albumin encapsulation, we are able to modulate RE biodistribution, improve the pharmacokinetics and magnify the accumulation of the REs in tumour tissue by >10-fold compared to uncoated REs. Thus, RE probes offer significant improvements over existing SWIR-emitting compounds by combining greater detection sensitivity, improved biological tolerance and multispectral imaging capabilities, underscoring the excellent potential for these nanomaterials for biomedical imaging applications. Preparation and characterization of multispectral REs REs were synthesized as core-shell structures consisting of a rare-earth-doped NaYF 4 core surrounded by an undoped NaYF 4 shell ( Fig. 1a ). REs displayed uniform spherical morphologies and narrow size distributions (~10–12 nm) that were confirmed by TEM micrographs ( Fig. 1b ). By doping the NaYF 4 core with ytterbium (Yb) and one of several other rare-earth elements, such as erbium (Er), holmium (Ho), thulium (Tm) or praseodymium (Pr) ( Supplementary Fig. S1 ), the emission properties of REs can be tailored in both the SWIR ( Fig. 1c ) and visible ( Supplementary Fig. S2 ) ranges. The fluorescence of REs occurs following the resonant transfer of excitation energy from a sensitizer (Yb) to an activator dopant such as Er, Ho, Tm or Pr [18] , [19] . The relaxation from an excited state results in the generation of SWIR emissions that are unique to the specific rare-earth activator ( Fig. 1d ). Hexagonal-phase, NaYF 4 , Yb:Er nanoparticles (REs) ( Fig. 1e ) were among the brightest SWIR-emitting rare earth-doped phosphors ( Fig. 1f ), and therefore were chosen to illustrate both the benefits of SWIR compared to conventional optical imaging methods as well as the biomedical potential for SWIR-based imaging approaches [19] , [20] . Compared to other SWIR emitters, the REs presented in this work are considerably more effective at generating SWIR emissions than SWNTs and IR-26, an organic SWIR dye ( Supplementary Fig. S3 ). Only highly toxic, lead-based QDs [10] , [21] , [22] matched the SWIR emission power output of the REs. 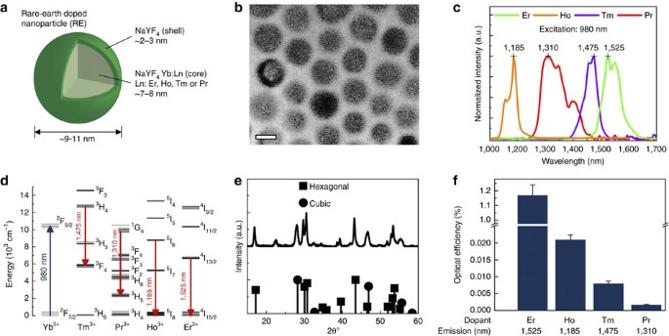Figure 1: Properties of the rare-earth-doped nanoprobes. (a) Rare earth nanoprobes consist of a NaYF4Yb:Ln-doped core (Ln: Er, Ho, Tm or Pr) surrounded by an undoped shell of NaYF4. TEM images of nanoprobes (b) show uniform 10-nm spherical particles (scale bar=10 nm). SWIR emissions can be tuned (c) by selecting suitable rare earth ion emitting centres. Probes consisting of a NaYF4host doped with ytterbium (Yb) and one or more elements selected from holmium (Ho), praseodymium (Pr), thulium (Tm) and erbium (Er) enable emissions at 1185, 1310, 1475 and 1525, nm, respectively. The 1185, 1310, 1475 and 1525, nm emissions of Ho-, Pr-, Tm- and Er-doped samples are attributed to the5I6→5I8,1G4→3H5,3H4→3F4, and4I13/2→4I15/2transitions, respectively (d). X-ray diffraction (XRD) plot (e) of nanoprobes confirm a predominately hexagonal-phase crystalline structure. The ranking for the optical efficiencies (f) of the differently doped systems is Er>Ho>Tm>Pr, where the relative ratios are 688:12:5:1, respectively. Bar graph data are expressed as mean values±standard deviation (s.d.);n=3. Figure 1: Properties of the rare-earth-doped nanoprobes. ( a ) Rare earth nanoprobes consist of a NaYF 4 Yb:Ln-doped core (Ln: Er, Ho, Tm or Pr) surrounded by an undoped shell of NaYF 4 . TEM images of nanoprobes ( b ) show uniform 10-nm spherical particles (scale bar=10 nm). SWIR emissions can be tuned ( c ) by selecting suitable rare earth ion emitting centres. Probes consisting of a NaYF 4 host doped with ytterbium (Yb) and one or more elements selected from holmium (Ho), praseodymium (Pr), thulium (Tm) and erbium (Er) enable emissions at 1185, 1310, 1475 and 1525, nm, respectively. The 1185, 1310, 1475 and 1525, nm emissions of Ho-, Pr-, Tm- and Er-doped samples are attributed to the 5 I 6 → 5 I 8 , 1 G 4 → 3 H 5 , 3 H 4 → 3 F 4 , and 4 I 13/2 → 4 I 15/2 transitions, respectively ( d ). X-ray diffraction (XRD) plot ( e ) of nanoprobes confirm a predominately hexagonal-phase crystalline structure. The ranking for the optical efficiencies ( f ) of the differently doped systems is Er>Ho>Tm>Pr, where the relative ratios are 688:12:5:1, respectively. Bar graph data are expressed as mean values±standard deviation (s.d. ); n =3. Full size image Tissue transmittance of SWIR emissions from REs To demonstrate the benefits of SWIR compared to wavelengths traditionally used for optical imaging, the absorbance, scattering and penetration depth properties of SWIR, NIR and visible light were evaluated in biological and phantom tissues. In biological tissues such as the skin, both blood haemoglobin and melanin pigment act as the primary chromophores or absorbers of light. [5] To quantify the improved tissue transmittance of SWIR, we used an integrating sphere to measure the attenuation of both SWIR and visible light after passing through blood and melanin-rich tumour tissue samples. SWIR light at 1,525 nm transmits three- and two-times more effectively in oxygenated blood and melanin-containing tumours, respectively, than 550 nm light ( Fig. 2a ). 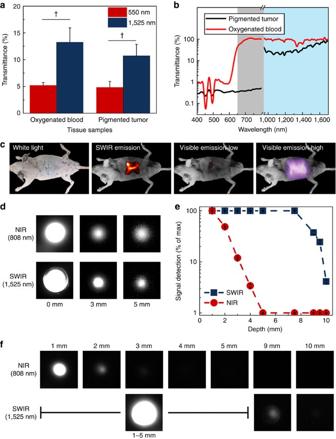Figure 2: RE nanoprobe SWIR tissue transmission is superior to that of NIR and visible light. SWIR light (1525, nm) emitted from Er-doped REs is significantly more effective at transmitting through blood and pigmented tumour tissue (a) than visible light at 550 nm. Bar graph data in (a) are expressed as mean values±standard error (s.e.m.);n=3 (†P<0.01) determined by Student’st-test. Transmission spectra (b) of visible (white region), NIR (grey region) and SWIR (blue region) light reveal that SWIR wavelengths exhibit lower absorbance and improved transmission through strong tissue absorbers such as blood and pigmented tumor tissue. Note the break in the spectra from 800 to 900 nm is due to the spectrometer’s detector change. The SWIR emissions from REs patterned into the shape of an ‘R’ and irradiated with 980 nm light (‘low’—0.14 W cm−2; ‘high’—0.5 W cm−2) were more clearly visualized through a mouse body (c) and at lower power densities than visible emissions due to reduced scattering and absorbance. Tissue phantom studies (d) comparing scattering from 808 nm NIR to 1525, nm SWIR light demonstrate improved resolution quality of SWIR signals. The intensities of both the SWIR and NIR light were measured to be identical prior to the application of the tissue phantoms. Signal intensity of SWIR and NIR light as a function of tissue phantom depth (e) shows complete attenuation of NIR light by 5 mm, whereas SWIR light is able to be detected through 10 mm of phantom tissues (f). Data in (f) are expressed as mean values±s.d.;n=3. The power outputs from the SWIR and NIR sources were adjusted to be identical (~30 μW) before tissue phantoms were applied. Figure 2: RE nanoprobe SWIR tissue transmission is superior to that of NIR and visible light. SWIR light (1525, nm) emitted from Er-doped REs is significantly more effective at transmitting through blood and pigmented tumour tissue ( a ) than visible light at 550 nm. Bar graph data in ( a ) are expressed as mean values±standard error (s.e.m. ); n =3 († P <0.01) determined by Student’s t -test. Transmission spectra ( b ) of visible (white region), NIR (grey region) and SWIR (blue region) light reveal that SWIR wavelengths exhibit lower absorbance and improved transmission through strong tissue absorbers such as blood and pigmented tumor tissue. Note the break in the spectra from 800 to 900 nm is due to the spectrometer’s detector change. The SWIR emissions from REs patterned into the shape of an ‘R’ and irradiated with 980 nm light (‘low’—0.14 W cm −2 ; ‘high’—0.5 W cm −2 ) were more clearly visualized through a mouse body ( c ) and at lower power densities than visible emissions due to reduced scattering and absorbance. Tissue phantom studies ( d ) comparing scattering from 808 nm NIR to 1525, nm SWIR light demonstrate improved resolution quality of SWIR signals. The intensities of both the SWIR and NIR light were measured to be identical prior to the application of the tissue phantoms. Signal intensity of SWIR and NIR light as a function of tissue phantom depth ( e ) shows complete attenuation of NIR light by 5 mm, whereas SWIR light is able to be detected through 10 mm of phantom tissues ( f ). Data in ( f ) are expressed as mean values±s.d. ; n =3. The power outputs from the SWIR and NIR sources were adjusted to be identical (~30 μW) before tissue phantoms were applied. Full size image We further investigated the attenuation properties of actual biological tissues in the SWIR by measuring the absorbance spectra of excised tissues obtained from a mouse exhibiting pigmented tumour lesions. The majority of tissue samples exhibit markedly low attenuation between 1,000–1,350 nm as well as between 1,500–1,650 nm, effectively extending the wavelength region of lowered attenuation within the second ‘tissue-transparent window’ of SWIR ( Supplementary Fig. S4 ) [8] , [12] . Furthermore, strong tissue absorbers like melanin in tumour samples, and haemoglobin in blood samples exhibited strong attenuation in the visible regime while attenuation in the SWIR was weak ( Fig. 2b ). Importantly, <0.4% of NIR light penetrated through 0.5 cm of pigmented tumour tissue compared to ~80% transmittance achieved by SWIR, suggesting NIR has limited use for detecting optical probes in tissues containing melanin. We demonstrated the imaging advantages afforded to SWIR due to the reduced tissue absorbance and scattering within this second window by patterning and depositing REs in the shape of an ‘R’ on a rubber mat beneath a mouse with resected intestines. When irradiated with low NIR excitation power (0.14 W cm −2 ), the visible emission from REs was not discernible, likely due to absorbance attenuation, while the ‘R’ pattern was clearly resolved by capturing the SWIR emission ( Fig. 2c ). Visible light could be detected through the mouse tissue when the excitation power was raised to 0.5 W cm −2 , but the resulting light scattering obscured the finer details of the ‘R’ pattern. To visualize the reduced scattering of SWIR relative to NIR, a pellet of REs was excited at 980 nm and the 1,525 nm signal was imaged using a portable InGaAs camera through increasing thickness of tissue phantoms composed of agarose and Intralipid, a common scattering agent [23] ( Supplementary Fig. S5 ). In comparison, an 808 nm source was used to simulate the standard emission wavelength of many NIR probes commonly used in biomedical imaging, such as indocyanine green [4] . By adjusting the output power of the 808 nm source and the excitation power used on the RE pellet, the intensities of both the SWIR emission and NIR source were measured to be identical by the InGaAs camera image analysis software prior to the application of the tissue phantoms. While the images captured at both wavelengths progressively lost focus with increasing phantom thickness, the SWIR signal was more distinct at greater depth ( Fig. 2d ). We determined the actual tissue penetration depth of SWIR compared to the current standard imaging wavelength region by measuring the intensity of SWIR and NIR light through tissue phantoms composed of both scattering and absorbing agents ( Supplementary Fig. S6 ). As before, images from the InGaAs camera were used to compare the penetration depth of the 808 nm NIR source and 1,525 nm SWIR-emitting RE pellet. In order to accurately compare the penetration depth of SWIR to NIR, the emitted power of the RE pellet and the output power of the NIR source were first matched to be identical (~30 μW) prior to the application of the tissue phantoms. The intensity of the NIR signal rapidly diminishes over increasing phantom depth with complete signal loss occurring by 5 mm ( Fig. 2e ). In contrast, the high SWIR emission from the RE pellet saturates the camera’s detector for phantom tissues ⩽ 5 mm. Notably, SWIR signal was detectable through 1 cm of phantom tissue, whereas no signal above background was seen using NIR ( Fig. 2f ). It is important to note that the 980 nm light used for exciting the RE pellet was not detectable by the camera through the use of appropriate filters. Although these results provide evidence for the significant advantages SWIR offers in biomedical imaging, in an actual imaging scenario light will need to penetrate through multiple tissue layers, resulting in refractive index changes that will lead to greater scatter [24] and lower signal-to-background ratios in the visible and NIR regimes than in the SWIR—further highlighting the benefits of SWIR. Biomedical application of SWIR-based imaging using REs As an emerging modality, SWIR-based imaging requires the design and implementation of a high-resolution system that can exploit SWIR capabilities for preclinical or clinical translation. Our portable in vivo imaging prototype [25] utilizes low energy density NIR light excitation well below the laser exposure limit for skin (defined as 0.73 W cm −2 for 980 nm) [26] and is capable of high-resolution, video-frame-rate SWIR image capture ( Fig. 3a ). Using a series of image processing algorithms ( Supplementary Fig. S7 ), SWIR signal intensities as a function of RE concentration were found to exhibit a linear relationship in both tissue phantoms and subcutaneous injections within mice, with a detection threshold at ~3 nM REs at an excitation power density of 0.14 W cm 2 and camera exposure time of ~50 ms per frame ( Supplementary Fig. S8 ). In comparison to QDs and SWNTs with reported detection limits of ~5 nM [27] and 6 nM [11] , respectively, REs can be detected at a lower concentration under comparable excitation. We evaluated the capabilities of this system to address several important optical imaging challenges including real-time probe detection and tracking, complex anatomical imaging of features at micrometre resolution and multispectral SWIR imaging of optical probes. 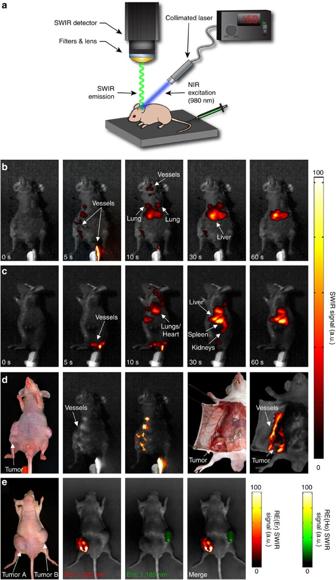Figure 3: RE nanoprobes enable real-time and multispectral imagingin vivo. Schematic of the portable SWIR-imaging prototype (a). The prototype consists of a room temperature-cooled InGaAs camera operating at a typical exposure time of 50 ms, adjustable filter mounts, a collimated laser with an output power density of 0.14 W cm−2and a neoprene rubber imaging surface. Real-time, video-rate biodistribution of intravenously injected REs captured in hairless mice using the imaging system prototype from both ventral (b) and left lateral (c) aspects. Nude mice bearing melanoma xenografts were intravenously injected with REs and imaged near surrounding tumor regions before dissection (d) from the ventral aspect. Proof-of-concept multiplexed SWIR imaging performed from the dorsal aspect in mouse xenografts (e) after Er- and Ho-doped rare-earth probes were separately injected into tumor sites on either flank of the animal. Representative images (n=3) are shown in all instances. Figure 3: RE nanoprobes enable real-time and multispectral imaging in vivo . Schematic of the portable SWIR-imaging prototype ( a ). The prototype consists of a room temperature-cooled InGaAs camera operating at a typical exposure time of 50 ms, adjustable filter mounts, a collimated laser with an output power density of 0.14 W cm −2 and a neoprene rubber imaging surface. Real-time, video-rate biodistribution of intravenously injected REs captured in hairless mice using the imaging system prototype from both ventral ( b ) and left lateral ( c ) aspects. Nude mice bearing melanoma xenografts were intravenously injected with REs and imaged near surrounding tumor regions before dissection ( d ) from the ventral aspect. Proof-of-concept multiplexed SWIR imaging performed from the dorsal aspect in mouse xenografts ( e ) after Er- and Ho-doped rare-earth probes were separately injected into tumor sites on either flank of the animal. Representative images ( n =3) are shown in all instances. Full size image We assessed the real-time in vivo SWIR-imaging capabilities of our prototype by intravenously injecting a bolus of REs into nude mice via catheterized tail veins. Immediately following injection, SWIR emissions were first identified in the tail vein (5 s) before clearing the vasculature to enter the heart and lungs (10 s). The beating of the heart in the chest of the mouse was visualized by pulsing SWIR emissions captured in real-time ( Supplementary Movies S1–2 ). Over the course of 60 s, the SWIR signal became progressively more intense in organs such as the liver and spleen, which are part of the reticuloendothelial system that mediates nanoparticle ( Fig. 3b ). In contrast, the accompanying RE upconversion visible signal was notably absent, probably due to absorption and scattering losses caused by blood and tissue components. We evaluated the disease tracking potential of SWIR by injecting intravenously into nude mice with developed melanoma xenografts. Shortly after injection, irregular branching patterns of SWIR emission were seen near tumours, which upon dissection were shown to correspond to the surrounding vasculature near tumours ( Fig. 3d , Supplementary Movie S3 ). In contrast to vasculature imaging methods using SWNTs, our imaging system is capable of visualizing REs in circulation at comparable camera resolutions (320 × 240) but at exposure durations that are 20 × shorter, and without requiring complex modifications to the camera optics [11] . To highlight the use of our imaging system for multispectral SWIR imaging, REs emitting at two different wavelengths were separately injected directly into tumour sites on both flanks of nude mice with xenograft melanomas. The direct injections of REs into separate tumours within the same animal ensured precise knowledge of probe localization as well as provided a common background for both sets of signals. Using a single NIR 980 nm excitation source, Er- and Ho-doped rare earth probes were detected at SWIR emission wavelengths of 1,525 and 1,175 nm, respectively. Separate filters attached to the camera enabled the observation of these wavelengths in two separate tumours with no crosstalk ( Fig. 3e ). This is the first successful demonstration of real-time multispectral SWIR imaging for in vivo applications using two of the SWIR-emitting REs. Tumour imaging using bioactive, albumin-coated REs The extension of SWIR for relevant clinical imaging applications such as cancer detection requires a probe formulation capable of directed tissue distribution while exhibiting favourable biomedical properties. For this purpose, REs were encapsulated in FDA-approved HSA to form rare-earth albumin nanocomposites ((RE)ANCs) using solvent-induced controlled coacervation of HSA ( Fig. 4a ). Our previous work has characterized the physiochemical properties of the (RE)ANCs and demonstrated that encapsulating REs in albumin improves the aqueous solubility of the rare-earth nanoprobes [28] . 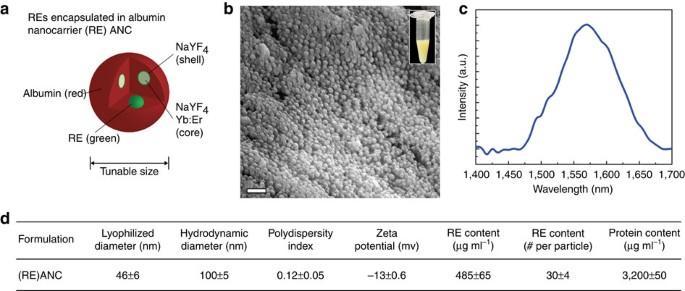Figure 4: Biologically permissive nanocomposites of REs exhibit SWIR emission. Rare-earth encapsulated albumin nanocarriers (RE(ANC)s) (a) consist of REs encapsulated by a coating of HSA to form an inorganic-organic nanocomposite, which can be tuned in size. SEM images (b) of (RE)ANCs show uniform sub-100 nm spherical particles (scale bar=200 nm). (RE)ANCs retain the SWIR emission of the encapsulated REs (c), exhibiting peak emission between 1550–1600, nm following 980 nm excitation. DLS measurements (d) confirm a low polydispersity and heterogeneity of size. (RE)ANCs exhibit negative zeta potentials in PBS (pH 7.4) and contain ~30 REs per particle. Data in (d) are expressed as mean values±s.d.;n=5. Figure 4c demonstrates that (RE)ANCs also retained the unique emission profile of the coated REs [29] . (RE)ANCs were fabricated at 100 nm hydrodynamic diameters and exhibited narrow polydispersity with slightly negative zeta potentials in PBS ( Fig. 4d ). The number of REs encapsulated per (RE)ANC was calculated to be ~30 REs per (RE)ANC using the viscosity/light scattering method [30] . Figure 4: Biologically permissive nanocomposites of REs exhibit SWIR emission. Rare-earth encapsulated albumin nanocarriers (RE(ANC)s) ( a ) consist of REs encapsulated by a coating of HSA to form an inorganic-organic nanocomposite, which can be tuned in size. SEM images ( b ) of (RE)ANCs show uniform sub-100 nm spherical particles (scale bar=200 nm). (RE)ANCs retain the SWIR emission of the encapsulated REs ( c ), exhibiting peak emission between 1550–1600, nm following 980 nm excitation. DLS measurements ( d ) confirm a low polydispersity and heterogeneity of size. (RE)ANCs exhibit negative zeta potentials in PBS (pH 7.4) and contain ~30 REs per particle. Data in ( d ) are expressed as mean values±s.d. ; n =5. Full size image To determine the biocompatibility of the rare-earth nanomaterials, the toxicity of REs and (RE)ANCs were evaluated in healthy, normal human epidermal melanocytes (NHEM). (RE)ANCs at all tested concentrations and REs <250 μg ml −1 did not significantly reduce cell viability ( Supplementary Fig. S9 ). These results support toxicity data from in vivo studies that have utilized REs for multiphoton upconversion visible imaging [31] , [32] . Furthermore, the FDA has approved the use of yttrium microspheres for the treatment of liver cancer, highlighting the long-term clinical translation potential of RE materials [33] . In contrast, SWIR-emitting PbS QDs have been shown to elicit adverse biological responses at concentrations as low as 20 μg ml −1 (ref. 21 ) and may undergo decomposition resulting in the release of toxic components under certain environmental conditions [22] . To assess tumour targeting and imaging capabilities, 10 nm REs and 100 nm (RE)ANCs ( Fig. 4d ) were separately injected intraperitoneally (IP) into transgenic (TGS) mice, an orthotopic melanoma model that spontaneously develops pigmented lesions that mimic the clinical progression of human melanoma [34] . The SWIR emission of (RE)ANCs in the peritoneal cavity progressively diminished over time, whereas emissions from the REs remain localized at the site of injection over 72 h ( Fig. 5a ). This is probably due to the aggregation of the non-encapsulated REs under aqueous conditions as previously reported [28] . All particle formulations appear to undergo clearance primarily through reticuloendothelial system organs ( Supplementary Fig. S10 ), which is characteristic of other nanomaterials including SWNTs [35] , [36] . The presence of yttrium in tissue samples was used as a marker for the particles. Detection of yttrium could be measured by inductively coupled plasma-mass spectrometry (ICP-MS) and correlated to particle concentration using a standard curve ( Supplementary Fig. S11 ). Pharmacokinetic data indicate that (RE)ANCs rapidly enter into circulation within 5 min after IP injection, while uncoated REs are not detectable at >0.05% injected dose g −1 within 6 h of injection ( Fig. 5b ). 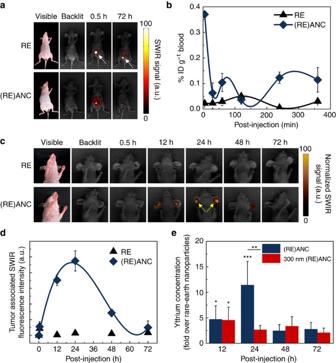Figure 5: RE biologic nanocomposites profile disease progressionin vivo. SWIR imaging of REs and (RE)ANCs after IP injection (a) into a transgenic orthotopic murine melanoma model (TGS) over 72 h. SWIR emission of non-encapsulated REs is observed localized in the abdominal cavity 0.5 h through 72 h post-injection (white arrows). Blood concentration (% injected dose per g) of yttrium (b) after RE and (RE)ANC IP injection. Data in (b) are expressed as mean values±s.e.m.;n=3. Tumor accumulation over time (c) of REs and (RE)ANCs in the ears of TGS mice after IP injection. Bright SWIR signal around the tumours was observed with (RE)ANCs (yellow arrows). Representative images (n=3) viewed from the ventral aspect are shown in all instances. The accumulation and clearance of SWIR fluorescence (d) in the tumours was described by a third-order polynomial fit for (RE)ANCs (R2=0.99) but could not be detected for REs. Data in (d) are expressed as mean values±s.d.;n=3. ICP-MS was performed (e) to detect the presence of yttrium in the tumours and quantify the imaging results observed in (c). Bar graph data are expressed as mean values±s.e.m.;n=10 for 12 h and 24 h,n=5 for 48 h and 72 h. *P<0.10; **P<0.05; ***P<0.02, determined by one-way ANOVA, Tukey post-hoc. Data in (e) are presented as a fold increase compared to REs. Figure 5: RE biologic nanocomposites profile disease progression in vivo . SWIR imaging of REs and (RE)ANCs after IP injection ( a ) into a transgenic orthotopic murine melanoma model (TGS) over 72 h. SWIR emission of non-encapsulated REs is observed localized in the abdominal cavity 0.5 h through 72 h post-injection (white arrows). Blood concentration (% injected dose per g) of yttrium ( b ) after RE and (RE)ANC IP injection. Data in ( b ) are expressed as mean values±s.e.m. ; n =3. Tumor accumulation over time ( c ) of REs and (RE)ANCs in the ears of TGS mice after IP injection. Bright SWIR signal around the tumours was observed with (RE)ANCs (yellow arrows). Representative images ( n =3) viewed from the ventral aspect are shown in all instances. The accumulation and clearance of SWIR fluorescence ( d ) in the tumours was described by a third-order polynomial fit for (RE)ANCs ( R 2 =0.99) but could not be detected for REs. Data in ( d ) are expressed as mean values±s.d. ; n =3. ICP-MS was performed ( e ) to detect the presence of yttrium in the tumours and quantify the imaging results observed in ( c ). Bar graph data are expressed as mean values±s.e.m. ; n =10 for 12 h and 24 h, n =5 for 48 h and 72 h. * P <0.10; ** P <0.05; *** P <0.02, determined by one-way ANOVA, Tukey post-hoc. Data in ( e ) are presented as a fold increase compared to REs. Full size image Furthermore, SWIR emissions from (RE)ANCs were observed at tumour sites near mouse ears between 12–48 h ( Fig. 5c ), with maximum emission observed at 24 h after IP injection ( Fig. 5d ), in agreement with other studies investigating nanoparticle accumulation in tumours after IP injection [37] , [38] . In contrast, REs did not distribute to the lesions over 72 h and were observed at the site of injection even after 144 h (data not shown). In addition, these results highlight the long-term in vivo stability of SWIR emission from REs. Our results present the first evidence of SWIR imaging being used for identifying diseased tissue in an animal model using our uniquely formulated, biocompatible SWIR-emitting (RE)ANCs. Notably, our imaging studies revealed no significant sources of non-specific tissue autofluorescence in the SWIR, confirming the low absorbance of SWIR observed in ex vivo tissue samples ( Supplementary Fig. S4 ) and the high signal-to-background ratios afforded to SWIR. To validate the distribution of SWIR fluorescence captured by the imaging system using a non-optical technique, we performed quantitative biodistribution studies to detect the presence of yttrium in tissue samples following RE and RE(ANC) injection using ICP-MS. We confirmed that (RE)ANCs exhibit enhanced accumulation at tumour sites by 12 h and are present at over 10-fold higher concentration than REs by 24 h ( Fig. 5e ). The accumulation of the (RE)ANCs at tumour sites may be due both to albumin-mediated active transport into the tumour interstitial space [39] and to the enhanced permeation and retention effect mediated by endothelial cells lining blood vessels near tumours. The enhanced permeation and retention effect enables nanoparticles on the order of 100 nm to leak from blood plasma and accumulate in tumour tissue [29] , [40] . To investigate the impact of the albumin coating on the tumour accumulation of encapsulated REs, (RE)ANCs with a larger HSA coating (~300 nm) ( Supplementary Fig. S12 ) were synthesized and the particle biodistribution tracked after injection into TGS mice ( Supplementary Fig. S10 ). Compared to the other sizes of nanoparticles used in this study ( Supplementary Fig. S13 ), the 300 nm (RE)ANCs exhibited reduced accumulation and retention at lesion sites ( Fig. 5e , Supplementary Fig. S14 ), highlighting the importance of both size and surface characteristics for influencing probe accumulation. Despite the exceptional optical imaging capabilities offered by the SWIR spectral region compared to traditional imaging in the visible and NIR regions, the development of materials that can harness and effectively utilize SWIR for biomedical applications has been limited. In comparison to other biomedical imaging modalities, optical imaging offers greater detection sensitivity, rapid real-time imaging using non-ionizing radiation and the ability to visualize multiple biological features simultaneously by using a variety of signals. Current SWIR probes have been unable to leverage these advantages to demonstrate the full potential of SWIR-based optical imaging for biomedical applications. To address this critical need, we have developed non-toxic, brightly emitting REs that are tunable over the entire SWIR region and evaluated the performance of these probes for biomedical imaging applications. By using a panel of RE probes, we are the first to demonstrate real-time and multispectral SWIR tissue imaging. REs were capable of resolving anatomical structures including organs, tumours and blood vessels using video-rate SWIR-imaging at micrometre resolution and millimetre depths. REs have been shown to be capable of molecular-level imaging [28] , and our current work extends the versatility of REs for use in real-time imaging of physiological features, such as the circulatory system, by exploiting the exceptional tissue transmission of SWIR. In addition to blood, our results indicate that SWIR is much more efficient than NIR or visible light at penetrating tissues with high concentrations of melanin and thus expanding the use of SWIR for noninvasive imaging through various skin types. Critically, we are the first to show in vivo SWIR imaging of diseased lesions using REs modified to target melanoma. By encapsulating REs via surface modification with FDA-approved albumin, we were able to improve the bioactivity of the REs, leading to enhanced RE accumulation at tumours that resulted in localized SWIR signal amplification and detection. The encapsulation of REs using albumin yields differentially sized composites and offers an alternative approach of modulating the bioactivity of other inorganic particles such as QDs, magnetic and gold nanoparticles to improve tumour accumulation. Furthermore, albumin offers functional groups for conjugating biomarker-specific targeting agents [28] as well as drug-binding sites that can be used to carry therapeutic agents [41] . Thus, this work provides a library of tunable, biocompatible rare-earth doped-nanomaterials as probes alongside a platform imaging technology suitable for a wide variety of biomedical applications including real-time nanomaterial tracking, deep tissue imaging and cancer lesion detection and monitoring. Synthesis of rare earth nanoprobes NaYF 4 :Yb-Ln (Ln=erbium (Er), holmium (Ho), praseodymium (Pr) and thulium (Tm)) nanoprobe powders were prepared using either a solvothermal decomposition or hydrothermal method (see Supplementary Methods ). Er-doped nanoprobes (REs) used for albumin encapsulation and in vivo imaging studies were synthesized through solvothermal decomposition [28] . Rare earth probes used for optical measurements were synthesized using a hydrothermal process [42] . Physical, chemical and optical characterization of rare earth nanoprobes Energy-dispersive X-ray spectroscopy area scan measurements of powder samples were made using the field emission scanning electron microscope (Carl Zeiss Σigma, Peabody, MA, USA) at 25 kV with a working distance of 8.5 mm for an aperture of 30 μm. The energy-dispersive X-ray elemental composition was determined by comparing relative peak intensities together with the corresponding sensitivity factors of each element and assuming their total intensities to be 100%. The emission spectra of powder samples in a 0.5-cm path length cell were recorded following excitation using a 2.5-W 975-nm photodiode (model BWF-OEM 975, BW Tek, Newark, NJ, USA). The emission from the sample was collected using a FSP920 spectrometer (Edinburgh Instruments, Livingston, UK) that was equipped with a Hamamatsu G5852-23 thermoelectrically cooled SWIR-sensitive indium gallium arsenide (InGaAs) photodiode. Optical efficiency measurements were performed using a modification of the C9220-03 quantum yield measurement system (Hamamatsu, Bridgewater, NJ, USA) [20] (see Supplementary Methods ). REs were visualized by using a transmission electron microscope (TEM) (JEOL 2010F, Tokyo, Japan) operated at 200 kV (see Supplementary Methods ). Optical measurements of tissue attenuation and scattering The scattering of 1,525 nm and 808 nm light was captured with a thermoelectric-cooled InGaAs SWIR camera (Goodrich, Princeton, NJ, USA) with a detection range from 800 to 1,700 nm fitted with a 25 mm focal length SWIR Lens (StingRay Optics, Keene, NH, USA). 975 nm light from a photodiode coupled to a 600-μm fibre optic cable was placed directly underneath a 2-cm pellet of REs to generate 1,525 nm emission for imaging through increasing depths of phantoms made from 1% agarose and 1% Intralipid. Parallel experiments were performed with 808 nm light emitted from a 600 μm fibre optic cable coupled to a 808 nm photodiode (BW Tek). 1,100 nm longpass and 850 nm shortpass filters (ThorLabs, Newton, NJ, USA) were used for the SWIR and NIR measurements, respectively. Both SWIR and NIR signals were adjusted to similar intensities before phantoms were applied. To determine the depth of penetration, the attenuation of 1,525 nm and 808 nm light was captured with a thermoelectric-cooled InGaAs SWIR camera (Goodrich, Princeton, NJ) with a detection range from 800 to 1,700 nm fitted with a 25-mm focal length SWIR Lens (StingRay Optics). Collimated 975 nm light was introduced directly underneath a 2-cm pellet of REs to generate 1,525 nm emission. Imaging was then performed through increasing the depths of phantoms made from 1% agarose, 1% Intralipid (Sigma-Aldrich, Milwaukee, WI, USA) and 0.1% India ink (Speedball Super Black, Statesville, NC, USA). Parallel experiments were performed with 808 nm light emitted from a 600-μm fibre optic cable coupled to a 808 nm photodiode (BW Tek). The power of the 808 nm source was adjusted to ~30 μW to match the power output at 1,525 nm from the RE pellet. 850 nm shortpass and 1,100 nm longpass filters (ThorLabs) were installed in the InGaAs camera to capture the NIR and SWIR light, respectively. Measurements were made in triplicate and quantified by mean intensity within a region of interest collected using the camera software. Absorption measurements of biological tissues were conducted using a double-beam spectrophotometer (Perkin-Elmer Lambda 9, Wellesley, MA, USA). Samples in 0.5-cm cuvettes were mounted in the path of the incoming beam. Following perfusion, various biological tissue samples including liver, spleen, kidneys, lungs, heart, brain, muscle, fat, bone, skin, peritoneum cavity and tumours were taken from transgenic mice. All samples were rinsed and kept in phosphate-buffered saline (PBS) after harvesting. Blood samples were collected in ethylenediaminetetraacetic acid (EDTA) collection tubes for the analysis. All samples were left on ice and measurements were recorded within several hours of harvesting. For comparing resolution differences between SWIR and visible light, ~0.2 g of REs were patterned into an ‘R’ using multipurpose casein glue (Elmer’s, Westerville, OH, USA). TGS mice were killed and intestinal tracts removed to reduce interference with faecal matter. The patterned REs were placed below the animal and irradiated with 980 nm light. Images were captured with either an InGaAs camera with a 1,100 nm longpass and two 1,152 nm bandpass filters (ThorLabs) for SWIR images, or a silicon-based camera (Canon Powershot SD780IS, Lake Success, NY, USA) with a 900-nm shortpass filter (ThorLabs) for visible images. (RE)ANC synthesis and characterization (RE)ANCs were prepared through a controlled coacervation technique as described previously [28] (see Supplementary Methods ). The nanoparticles were concentrated by a factor of 10 using centrifugation (Beckman Coulter, Avanti J-E Centrifuge). Redispersion was performed in an ultrasonication bath (Fisher Scientific, FS60) for 15 min. (RE)ANCs size and surface characteristics from at least four separate batches of particles were measured and averaged using a Malvern Zetasizer Nano (Zen 3690, Malvern, Worcestershire, UK) (see Supplementary Methods ). (RE)ANCs were visualized with a scanning electron microscope (Carl Zeiss Σigma) operated at 5.0 kV with working distance of 10 mm using the secondary electron detector (see Supplementary Methods ). For number average size measurements, diameters of ~100 (RE)ANCs were measured from scanning electron microscope images. The number of REs in the (RE)ANCs was determined by the viscosity-light scattering method [30] (see Supplementary Methods ). Animal models Initial imaging studies were conducted using nude mice (Taconic, Hudson, NY, USA). Human melanoma cells, C8161 (Dr Mary J.C. Hendrix, Children’s Memorial Research Center, Chicago, IL, USA), were injected into the dorsal area at 10 6 cells per site. Biodistribution and tumour accumulation studies were performed using transgenic mice developed by Chen et al . [34] , which are predisposed to develop multiple melanomas (TG-3). As described previously, these transgenic mice develop spontaneous melanin-containing dermal lesions in the absence of any known carcinogen or ultraviolet radiation in as early as 10–12 days. Hairless TG-3, also referred to as TGS, were developed for ease of tumour visualization and were used in this study. The animals were inspected and graded for tumour development twice weekly. Animals were used for imaging and biodistribution studies once lesion thickness reached 1 mm on the ears. All animal studies were approved by the Institutional Review Board for Animal Care and Facilities Committee of Rutgers University and performed in accordance with institutional guidelines on animal handling. Proof-of-concept in vivo imaging An in-house prototype of a small-animal SWIR-imaging system was utilized to investigate the use of the nanocomposites for noninvasive fluorescence imaging (see Supplementary Methods ). Real-time SWIR imaging was performed in nude mice and vascular SWIR imaging was performed in xenograft mice. Catheters consisting of polyethylene tubing (Becton, Dickinson and Company, Sparks, MD, USA) were implanted into the tail veins and secured to tongue depressors. A bolus of ~200 μl of 2 mg RE nanoprobes per ml was slowly infused over 5 s while the mouse was continuously scanned with collimated 980 nm laser light. Five-second segmented clips of the recorded SWIR videos were used for post-processing. Multiplex imaging of Er- and Ho-doped rare earth probes was performed in xenograft mice after an intratumoral injection of 100 μl (2 mg particles per ml). To distinguish emissions from Er-doped formulation, a combination of one 1,400-nm longpass (FEL1400, ThorLabs) and two 1,550-nm (FB1550-12, ThorLabs) bandpass filters was used, while a 1,100-nm longpass (FEL1100, ThorLabs) and two 1,152-nm bandpass filters (FL1152-10, ThorLabs) were used to identify the Ho-doped formulation. Videos were also subjected to post-processing as discussed. Qualitative biodistribution imaging TGS mice were fully anesthetized with an intraperitoneal injection (IP) of Avertin (240 mg kg −1 ) (Sigma-Aldrich) prior to imaging. Mice were scanned with the collimated 980 nm laser prior to nanocomposite injection (background image). Mice were then injected via IP with either 10 mg kg −1 of uncoated REs, (RE)ANCs or 300 nm (RE)ANCs resuspended in PBS and normalized to RE content for all formulations. Mice were irradiated under anaesthesia with the collimated 980 nm laser in various positions at different post-injection time-points. Quantitative biodistribution analysis Mice exhibiting vascularized melanoma tumours were injected via IP with either 2 mg kg −1 of uncoated REs, (RE)ANCs or 300 nm (RE)ANCs resuspended in PBS and normalized to RE content for all formulations. At 24 h the mice were killed and their organs were collected, rinsed with PBS and weighed. Mice were housed in metabolic chambers for the collection of faeces. To quantify REs in circulation, blood was intermittently sampled through the tail vein. Samples were stored at −80 °C before acid digestion. The yttrium content of digested organs was quantified using a Thermo X series II ICP-MS (Thermo Scientific, Waltham, MA, USA) to determine particle concentration after injection (see Supplementary Methods ). How to cite this article: Naczynski, D. J. et al . Rare-earth-doped biological composites as in vivo shortwave infrared reporters. Nat. Commun. 4:2199 doi: 10.1038/ncomms3199 (2013).